Cluster synchronization and isolated desynchronization in complex networks with symmetries Synchronization is of central importance in power distribution, telecommunication, neuronal and biological networks. Many networks are observed to produce patterns of synchronized clusters, but it has been difficult to predict these clusters or understand the conditions under which they form. Here we present a new framework and develop techniques for the analysis of network dynamics that shows the connection between network symmetries and cluster formation. The connection between symmetries and cluster synchronization is experimentally confirmed in the context of real networks with heterogeneities and noise using an electro-optic network. We experimentally observe and theoretically predict a surprising phenomenon in which some clusters lose synchrony without disturbing the others. Our analysis shows that such behaviour will occur in a wide variety of networks and node dynamics. The results could guide the design of new power grid systems or lead to new understanding of the dynamical behaviour of networks ranging from neural to social. Synchronization in complex networks is essential to the proper functioning of a wide variety of natural and engineered systems, ranging from electric power grids to neural networks [1] . Global synchronization, in which all nodes evolve in unison, is a well-studied effect, the conditions for which are often related to the network structure through the master stability function [2] . Equally important, and perhaps more ordinary, is partial or cluster synchronization (CS), in which patterns or sets of synchronized elements emerge [3] . Recent work on CS has been restricted to networks where the synchronization pattern is induced either by tailoring the network geometry or by the intentional introduction of heterogeneity in the time delays or node dynamics [4] , [5] , [6] , [7] , [8] , [9] , [10] , [11] . These anecdotal studies illustrate the interesting types of CS that can occur, and suggest a broader relationship between the network structure and synchronization patterns. Recent studies have begun to draw a connection between network symmetry and CS, although all have considered simple networks where the symmetries are apparent by inspection [12] , [13] , [14] . More in-depth studies have been done involving bifurcation phenomena and synchronization in ring and point symmetry networks [15] , [16] . Finally, a form of CS can occur in situations where input and output couplings match in a cluster, but there is no symmetry [16] , [17] . Here we address the more common case where the intrinsic network symmetries are neither intentionally produced nor easily discerned. We present a comprehensive treatment of CS, which uses the tools of computational group theory to reveal the hidden symmetries of networks and predict the patterns of synchronization that can arise. We use irreducible group representations to find a block diagonalization of the variational equations that can predict the stability of the clusters. We further establish and observe a generic symmetry-breaking bifurcation termed isolated desynchronization, in which one or more clusters lose synchrony while the remaining clusters stay synchronized. The analytical results are confirmed through experimental measurements in a spatiotemporal electro-optic network. By statistically analysing the symmetries of several types of networks, as well as electric power distribution networks, we argue that symmetries, clusters and isolated desynchronization can occur in many types of complex networks and are often found concurrently. Throughout the text, we use the abbreviation ID for isolated desynchronization. The dynamical equations A set of general dynamical equations to describe a network of N -coupled identical oscillators are where x i is the n -dimensional state vector of the i th oscillator, F describes the dynamics of each oscillator, A is a coupling matrix that describes the connectivity of the network, σ is the overall coupling strength and H is the output function of each oscillator. Equation (1) or its equivalent forms provide the dynamics for many networks of oscillators, including all those in refs 1 , 2 , 3 , 4 , 6 , 7 , 8 , 11 , 12 , 13 , 14 . This includes some cases of time delays in the coupling functions. As noted in ref. 1 , it is only necessary for the form of the equations of motion or, more importantly, the variational equations to have the form of equation (1) near the synchronization manifolds. The form of equation (1) also applies to discrete time systems or more general coupling schemes [18] . In addition, the same form emerges in the more general case for the variational equations where the vector field and the coupling combine into one function, viz. F (x i ( t ), {x j (t)}), where the argument in brackets is the input of all nodes connected to node i , so long as the nodes are treated as having the same basic dynamics. See ref. 18 for more explanation. Generalizations of equation (1) have been studied in refs 5 , 9 , 10 , 19 . The types of natural and man-made systems, which can be modelled by equations of the same form as equation (1), are large [20] , [21] . These include genetic networks, circadian networks, ecology, neuronal networks, cortical networks, consensus problems, opinion formation, power grids and concentration of metabolites in a cell to name a few. The same analysis as presented here will apply to more general dynamics. Here, for simplicity, we take all nodes to have identical dynamics and be bidirectionally coupled to other nodes in the network by couplings of the same weight, that is, A ij is taken to be the (symmetric) adjacency matrix of 1’s and 0’s with the factor of σ controlling the weight of the couplings. The vector field F can contain self-feedback terms. Here we take the self-feedback to be identical for all nodes. The cases of Laplacian coupling schemes are encompassed by our analysis as shown here. This is because the row sums are not affected by the symmetry operations. Laplacian coupling schemes are often used to tune the network specifically for global synchronization, which is not our goal here. We think our scheme may be more representative of networks that form naturally (for example, neurons) where row sums will not necessarily appear in the feedback. The cases of directional (non-symmetric) coupling, variations of coupling weight and non-identical nodes can all be handled in much the same way as presented here, although it is not clear that those more general cases will have as many symmetries as our simpler case. The symmetries of the network form a (mathematical) group . Each symmetry g of the group can be described by a permutation matrix R g that re-orders the nodes in a way that leaves the dynamical equations unchanged (that is, each R g commutes with A ). The set of symmetries (or automorphisms) [15] , [22] of a network can be quite large, even for small networks, but it can be calculated from A using widely available discrete algebra routines [23] , [24] . 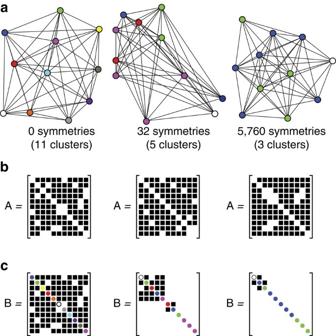Figure 1: Three randomly generated networks with varying amounts of symmetry and associated coupling matrices. (a) Nodes of the same colour are in the same synchronization cluster. The colours show the maximal symmetry the network dynamics can have given the graph structure. (b) A graphic showing the structure of the adjacency matrices of each network (black squares are 1, white squares are 0). (c) Block diagonalization of the coupling matrices A for each network. Colours denote the cluster, as ina. The 2 × 2 transverse block for the 32 symmetry case comes from one of the IRRs being present in the permutation matrices two times. The matrices for the 32 symmetry case are shown in the Methods section. Figure 1a shows three graphs generated by randomly removing 6 edges from an otherwise fully connected 11-node network. Although the graphs appear similar and exhibit no obvious symmetries, the first instance has no symmetries (other than the identity permutation), while the others have 32 and 5,760 symmetries, respectively. Thus, for even a moderate number of nodes (11), finding the symmetries can become impossible by inspection. Figure 1: Three randomly generated networks with varying amounts of symmetry and associated coupling matrices. ( a ) Nodes of the same colour are in the same synchronization cluster. The colours show the maximal symmetry the network dynamics can have given the graph structure. ( b ) A graphic showing the structure of the adjacency matrices of each network (black squares are 1, white squares are 0). ( c ) Block diagonalization of the coupling matrices A for each network. Colours denote the cluster, as in a . The 2 × 2 transverse block for the 32 symmetry case comes from one of the IRRs being present in the permutation matrices two times. The matrices for the 32 symmetry case are shown in the Methods section. Full size image Once the symmetries are identified, the nodes of the network can be partitioned into M clusters by finding the orbits of the symmetry group: the disjoint sets of nodes that when all of the symmetry operations are applied permute among one another [15] . As equation (1) is essentially unchanged by the permutations, the dynamics of the nodes in each cluster can be equal, which is exact synchronization. Hence, there are M synchronized motions {s 1 ,…, s M }, one for each cluster. In Fig. 1a , the nodes have been coloured to show the clusters. For the first example, which has no symmetries, the network divides into M = N trivial clusters with one node in each. The other instances have five and three clusters, respectively. Once the clusters are identified, equation (1) can be linearized about a state where synchronization is assumed among all of the nodes within each cluster. This linearized equation is the variational equation and it determines the stability of the clusters. The variational equations Equation (1) is expressed in the node coordinate system, where the subscripts i and j are identified with enumerated nodes of the network. Beyond identifying the symmetries and clusters, group theory also provides a powerful way to transform the variational equations to a new coordinate system in which the transformed coupling matrix B = TAT −1 has a block diagonal form that matches the cluster structure, as described below. The transformation matrix T is not a simple node re-ordering, nor is it an eigendecomposition of A . The process for computing T is non-trivial, and involves finding the irreducible representations (IRRs) of the symmetry group. We call this new coordinate system the IRR coordinate system. In the Methods section, we show the steps necessary to obtain the symmetries, clusters and the transformation T . Once we have T , we can transform the variational equations as follows. Let m be the set of nodes in the m th cluster with synchronous motion s m ( t ). Then, the original variational equations about the synchronized solutions are (in vectorial form and in the node coordinates), where the Nn -dimensional vector δ x ( t )=[ δ x 1 ( t ) T , δ x 2 ( t ) T ,..., δ x N ( t ) T ] T and E ( m ) is an N -dimensional diagonal matrix such that i =1,…, N . Note that , where I N is the N -dimensional identity matrix. Applying T to equation (2), we arrive at the variational matrix equation shown in equation (4), where η (t)= T ⊗ I n δ x ( t ), J ( m ) is the transformed E ( m ) and B is the block diagonalization of the coupling matrix A , where we have linearized about synchronized cluster states { s 1 ,..., s M }, η ( t ) is the vector of variations of all nodes transformed to the IRR coordinates, and D F and D H are the Jacobians of the nodes’ vector field and coupling function, respectively. We note that this analysis holds for any node dynamics, steady state, periodic, chaotic and so on. We can write the block diagonal B as a direct sum , where C l is a (generally complex) p l × p l matrix with p l =the multiplicity of the l th IRR in the permutation representation { R g }, L =the number of IRRs present and d ( l ) =the dimension of the l th IRR, so that (refs 25 , 26 ). For many transverse blocks, C l is a scalar, that is, p l =1. However, the trivial representation ( l =1), which is associated with the motion in the synchronization manifold has p 1 = M . Note that the vector field F can contain a self-feedback term β x i as in the experiment and other feedbacks are possible, for example, row sums of A ij , as long as those terms commute with the R g . In all these cases, the B matrix will have the same structure. Figure 1c shows the coupling matrix B in the IRR coordinate system for the three example networks. The upper-left block is an M × M matrix that describes the dynamics within the synchronization manifold. The remaining diagonal blocks describe motion transverse to this manifold and so are associated with loss of synchronization. Thus, the diagonalization completely decouples the transverse variations from the synchronization block and partially decouples the variations among the transverse directions. In this way the stability of the synchronized clusters can be calculated using the separate, simpler, lower-dimensional ODEs of the transverse blocks to see if the non-synchronous transverse behaviour decays to zero. 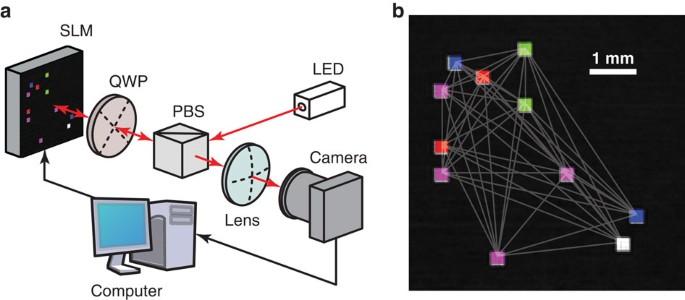Figure 2: Experimental configuration. (a) Light is reflected from the SLM and passes though polarization optics thus, that the intensity of light falling on the camera is modulated according the phase shift introduced by the SLM. Coupling and feedback are implemented by a computer. (b) An image of the SLM recorded by the camera in this configuration. Oscillators are shaded to show which cluster they belong to, and the connectivity of the network is indicated by superimposed grey lines. The phase shifts applied by the square regions are updated according to equation (5). An electro-optic experiment Figure 2a shows the optical system used to study cluster synchronization. Light from a 1,550-nm light-emitting diode passes through a polarizing beamsplitter and quarter wave plate, so that it is circularly polarized when it reaches the spatial light modulator (SLM). The SLM surface imparts a programmable spatially dependent phase shift x between the polarization components of the reflected signal, which is then imaged, through the polarizer, onto an infrared camera [27] . The relationship between the phase shift x applied by the SLM and the normalized intensity recorded by the camera is ( x )=(1−cos x )/2. The resulting image is then fed back through a computer to control the SLM. More experimental details are given in the Methods section. Figure 2: Experimental configuration. ( a ) Light is reflected from the SLM and passes though polarization optics thus, that the intensity of light falling on the camera is modulated according the phase shift introduced by the SLM. Coupling and feedback are implemented by a computer. ( b ) An image of the SLM recorded by the camera in this configuration. Oscillators are shaded to show which cluster they belong to, and the connectivity of the network is indicated by superimposed grey lines. The phase shifts applied by the square regions are updated according to equation (5). Full size image The dynamical oscillators that form the network are realized as square patches of pixels selected from a 32 × 32 tiling of the SLM array. Figure 2b shows an experimentally measured camera frame captured for 1 of the 11-node networks considered earlier in Fig. 1 (A full video is presented in the Supplementary Movie 1 ). The patches have been falsely coloured to show the cluster structure and the links of the network are overlaid to illustrate the connectivity. The phase shift of the i th region, x i , is updated iteratively according to: where β is the self-feedback strength and the offset δ is introduced to suppress the trivial solution x i =0. Equation (5) is a discrete time equivalent of equation (1). Depending on the values of β , σ and δ , equation (5) can show constant, periodic or chaotic dynamics. There are no experimentally imposed constraints on the adjacency matrix A ij , which makes this system an ideal platform to explore synchronization in complex networks. 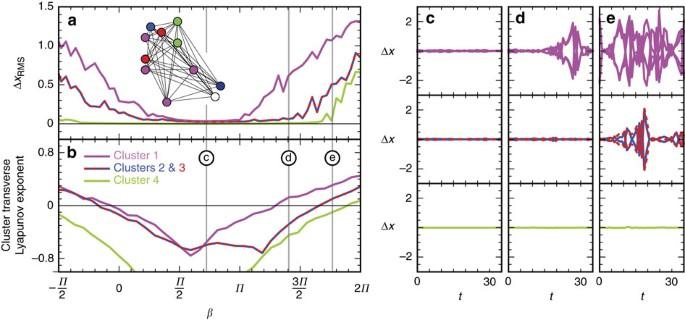Figure 3: Experimental observation of isolated and intertwined desynchronization. (a) CS error as the self-feedback,β, is varied. For all cases considered,δ=0.525 andσ=0.67π. Colours indicate the cluster under consideration and are consistent withFig. 1. (b) MLE calculated from simulation. (c–e) Synchronization error time traces for the four clusters, showing the isolated desychronization of the magenta cluster and the isolated desychronization of the intertwined blue and red clusters. Figure 3 plots the time-averaged root-mean square synchronization error for all four of the non-trivial clusters shown in Fig. 2b , as a function of the feedback strength β , holding σ constant. We find qualitatively similar results if σ is chosen as a bifurcation parameter with β held constant. In Fig. 3c–e , we plot the observed intracluster deviations for three specific values of β indicated by the vertical lines in Fig. 3a,b , showing different degrees of partial synchronization that can occur, depending on the parameters. Figure 3: Experimental observation of isolated and intertwined desynchronization. ( a ) CS error as the self-feedback, β , is varied. For all cases considered, δ =0.525 and σ =0.67 π . Colours indicate the cluster under consideration and are consistent with Fig. 1 . ( b ) MLE calculated from simulation. ( c – e ) Synchronization error time traces for the four clusters, showing the isolated desychronization of the magenta cluster and the isolated desychronization of the intertwined blue and red clusters. Full size image Details of the calculations are given in the Methods section. Supplementary Movie 1 illustrates the experimentally recorded network behaviour for the case of β =0.72 π , where the system clearly partitions into four synchronized clusters plus one unsynchronized node. Together, Fig. 3a,c–e illustrate two examples of a bifurcation commonly seen in experiment and simulation: isolated desynchronization, where one or more clusters lose stability, while all others remain synchronized. At β =0.72 π ( Fig. 3c ), all four of the clusters synchronize. At β =1.4 π ( Fig. 3d ), the magenta cluster, which contains four nodes, has split into two smaller clusters of two nodes each, while the other two clusters remain synchronized. Between β =0.72 π and β =1.767 π , two clusters, shown in Fig. 1 as red and blue, respectively, undergo isolated desynchronization together. In Fig. 3a , the synchronization error curves for these two clusters are visually indistinguishable. The synchronization of these two clusters is intertwined: they will always either synchronize together or not at all. Although it is not obvious from a visual inspection of the network that the red and blue clusters should form at all, their intertwined synchronization properties can be understood intuitively by examining the connectivity of the network. Each of the two nodes in the blue cluster is coupled to exactly one node in the red cluster. If the blue cluster is not synchronized, the red cluster cannot synchronize, because its two nodes are receiving different input. The group analysis treats this automatically and yields a transverse 2 × 2 block in Fig. 1c . The isolated desynchronization bifurcations we observe are predicted by computation of the maximum Lyapunov exponent (MLE) of the transverse blocks of equation (4), shown in Fig. 3 . The region of stability of each cluster is predicted by a negative MLE. Although there are four clusters in this network, there are only three MLEs: the two intertwined clusters are described by a two-dimensional block in the block-diagonalized coupling matrix B. These stability calculations reveal the same bifurcations as seen in the experiment. Subgroup decomposition and isolated desynchronization The existence of isolated desynchronizations in the network experiments raises several questions. As the network is connected why doesn’t the desynchronization pull other clusters out of sync? What is the relation of ID to cluster structure and network symmetry? Is ID a phenomenon that is common to many networks? We provide answers to all these questions using geometric decomposition of a group, which was developed in refs 28 , 29 . This technique enables a finite group to be written as a direct product of subgroups = 1 × ... × where is the number of subgroups and all the elements in one subgroup commute with all the elements in any other subgroup. This means that the set of nodes permuted by one subgroup is disjoint from the set of nodes permuted by any other subgroup. Then, each cluster (say, j ) is permuted only by one of the subgroups (say, k ), but not by any others. There can be several clusters permuted by one subgroup. This is the case of the red and blue clusters in the 32 symmetry network in Fig. 1 , because the associated k cannot have a geometric decomposition, but may have a more structured decomposition such as a wreath product [30] . We can show that the above decomposition guarantees that the nodes associated with different subgroups all receive the same total input from the other subgroups’ nodes. Hence, nodes of each cluster will not see the effects of individual behaviour of the other clusters associated with different subgroups. This enables the clusters to have the same synchronized dynamics even when another cluster desynchronizes. If that state is stable, we have ID. To see this let k , a subgroup of , permute only cluster m and π be the permutation on the indices of nodes in m for one permutation R g , g ε k . Assume x i is not in m ; thus, it is not permuted by R g and recall that A commutes with all permutations in , then we have (just concentrating on the terms from m ), where π ( l ) is, in general, another node in m and the sums over other clusters are unchanged. This shows that all nodes in m are coupled into the i th node in the same way (the same A ij factor). Similarly, if we use a permution R g′ on the cluster m′ containing x i , we can show that all the nodes of m are coupled in the same way to the nodes in m . Hence, nodes of m each receive the same input sum from the nodes of m whether the nodes of m are synchronized or not. This explains how the cluster m can become desynchronized, but the nodes of m can still be synchronized—they all have the same input despite the m desynchronization, thus making the m synchronous state flow invariant. If it is also stable, this is the case of ID. This argument is easily generalized to the case when k permutes nodes of several clusters as this will just add other similar sums to equation (6). The latter case explains the intertwined desynchronization in the experiment and is a more general form of ID. Symmetries for different network topologies How common is such an ID situation we outlined above? We have examined symmetry statistics for some classes of random and semi-random graph types, which suggest that when symmetries are present the opportunity for ID dynamics will be common, although the stability for such will depend on the dynamical systems of the network nodes. We emphasize that we are not attempting to compare symmetry statistics across different graph models, but only to generate networks that have different topologies (for example, random, tree-like and bipartite) to show common phenomena. We examined 10,000 realizations of three random and semi-random networks each with 100 nodes: (1) randomly connected nodes (random graphs) similar to Erdös–Renyi graphs [31] generated as described above but with 100 nodes and 50 random edges deleted; (2) scale-free (tree) graphs following Barabasi and Albert [32] , [33] ; and (3) random bipartite [23] graphs using the RandomBipartite function in Sage with 90 nodes in 1 partition and 10 in the other. Random graphs were generated by starting with 100 nodes completely connected and randomly deleting 50 edges. Scale-free Barabasi and Albert graphs were based on the original Barabasi and Albert preference algorithm [32] using the Sage routine RandomBarabasiAlbert. These had 100 nodes with 99 edges and a tree structure. Bipartite networks were generated with the Sage routine RandomBipartite ( n 1 , n 2 , p ), which generates a graph with two sets of nodes ( n 1 in the first partition and n 2 in the second partition, where n 1 + n 2 =100) and connections from nodes in the first partition to nodes in the second partition are added with probability p . We used n 1 =10, n 2 =90 and p =0.85. Ten thousand realizations of each graph type were generated. We tested several 10,000 realizations and we see very little variation in statistics between realizations of the same class leading us to believe that we are sampling fairly and enough to trust our results. We also checked for equivalent (isomorphic) graphs to see how much repetition we had. The random systems yielded on average 1 equivalent pair per 10,000 realizations. The scale-free cases yielded <0.01% equivalent graphs. Apparently, we are not near the maximum number of inequivalent graphs for any of the classes. Even with just 100 realizations, the main trends in number of symmetries and other statistics are evident, although such small samples occasionally miss those symmetry cases that are not too common in the class. 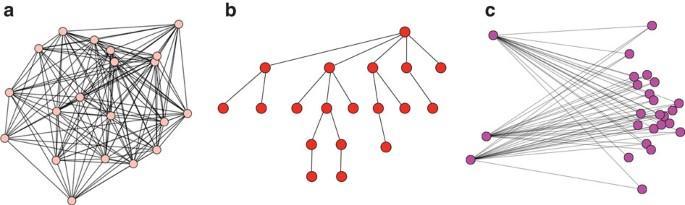Figure 4: Three graph topologies. Graph types analysed are (a) complete graph with random edges deleted, (b) Barabasi–Albert tree graphs and (c) bipartite graphs. The number of nodes shown is smaller (20–25) than the actual number used in the calculations (100) so that the topological structure of each type is clear. Figure 4 shows the different topologies of the networks. 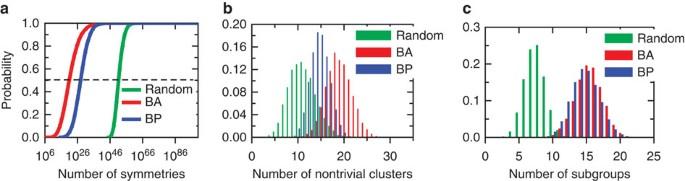Figure 5: Symmetry, cluster and subgroup statistics for three types of networks. The networks are random, Barabasi and Albert (BA in the figure), and the bipartite case (BP in the figure). The statistics are (a) the cumulative distribution of the number of symmetries (the dashed line is the median), (b) the counts of the number of non-trivial clusters and (c) the counts of the number of subgroups in the decomposition. The statistics were calculated using 10,000 realizations of each network. Figure 5a shows the cumulative distribution of symmetries for each type of network. All have similar distributions overall, but on different scales of symmetries. Almost all graphs for each type have several non-trivial clusters and more than one subgroup. The median numbers of clusters for the random, Barabasi and Albert, and bipartite networks are 11, 19 and 15, respectively. The median numbers of subgroups are 8, 15 and 15, respectively. The per cent of cases where the number of subgroups is less than the number of clusters (intertwined cases) are 98.45, 98.48 and 0%, respectively. Thus, in these networks symmetries, clusters and subgroups are simultaneously present and, thus, so is the scenario for ID. Figure 4: Three graph topologies. Graph types analysed are ( a ) complete graph with random edges deleted, ( b ) Barabasi–Albert tree graphs and ( c ) bipartite graphs. The number of nodes shown is smaller (20–25) than the actual number used in the calculations (100) so that the topological structure of each type is clear. Full size image Figure 5: Symmetry, cluster and subgroup statistics for three types of networks. The networks are random, Barabasi and Albert (BA in the figure), and the bipartite case (BP in the figure). The statistics are ( a ) the cumulative distribution of the number of symmetries (the dashed line is the median), ( b ) the counts of the number of non-trivial clusters and ( c ) the counts of the number of subgroups in the decomposition. The statistics were calculated using 10,000 realizations of each network. Full size image We also studied symmetries, clusters and subgroup decompositions in small-world graphs. Small-world graphs [31] , [34] were generated by starting with a ring of nearest-neighbour connected nodes, then adding a fixed number of edges to give the same number of edges as the random graphs in the text. We found we had to add many edges beyond the usual few used to generate the small-world effect, because adding only a few edges beyond the ring rarely resulted in any symmetries. As a result, the small-world examples approached being similar to the random graphs so we do not display their results, although the two systems each have symmetries that the other does not; hence, they appear to not be exactly identical. Finally, we examined some man-made and natural networks. The man-made networks are the Nepal power grid [35] and the Mesa del Sol electrical grid [36] . We show the Nepal grid, as its small size is easier to display in Fig. 6 . In addition, shown is the block diagonalization of the coupling matrix. Here we treat the grid analogous to ref. 1 in which all power stations are identical with the same bidirectional coupling along each edge which fits the model in equation (1). In this model, global synchronization (the usual desired state) is a solution of the equations of motion. However, as we have pointed out, if symmetry induced clusters exist, CS is also a solution of the equations of motion. The Nepal network has 86,400 symmetries, three non-trivial clusters (plus two trivial ones) and three subgroups (one for each nontrivial cluster). This implies it is possible for this network to split into three sets of synchronized clusters. This also implies that depending on the exact dynamics, the parameters and the stability of global and cluster states, it is possible that the CS state may be a route to desynchronization of the global state in the Nepal grid or other grids with similar dynamics. 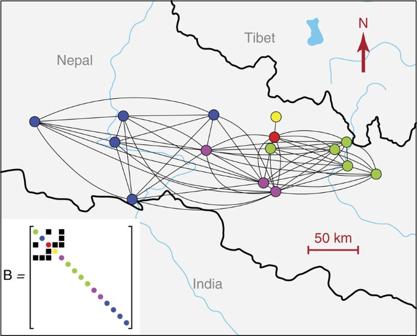Figure 6: Geographical diagram of the Nepal power grid network. Colours are used to indicate the computed cluster structure. The matrix (inset) shows the structure of the diagonalized coupling matrix, analogous toFig. 1a. The diagonal colours indicate which cluster is associated with each column. Figure 6: Geographical diagram of the Nepal power grid network. Colours are used to indicate the computed cluster structure. The matrix (inset) shows the structure of the diagonalized coupling matrix, analogous to Fig. 1a . The diagonal colours indicate which cluster is associated with each column. Full size image The Mesa del Sol electric grid has 4,096 symmetries, 20 non-trivial clusters and 10 subgroups. The network has three intertwined clusters, two with four clusters and one with five clusters. This is shown in Fig. 7 a circle plot of the Mesa del Sol network, which, because of the network size (132 nodes), exposes the cluster structure much better. As the Nepal example indicates, the symmetry structure makes global synchronization, CS and ID a possibility in the Mesa del Sol network. We note that the foregoing analysis of symmetries considers only the topology of the network. The dynamics of real electrical power networks is better described by a complex admittance matrix, for which the symmetries may be different. 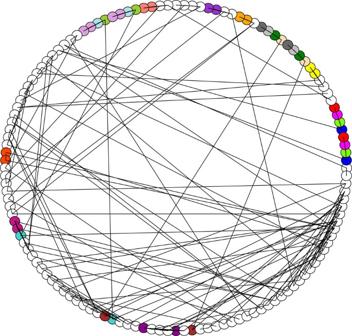Figure 7: Network and cluster structure of the Mesa del Sol electric grid. Colours are used to denote clusters. Nodes coloured white are trivial clusters, containing only one element. Figure 7: Network and cluster structure of the Mesa del Sol electric grid. Colours are used to denote clusters. Nodes coloured white are trivial clusters, containing only one element. Full size image Many other networks were studied for symmetries in refs 28 , 29 for the purpose of finding motifs and redundancies, but not dynamics. Those networks were Human B Cell Genetic Interactions, Caenorabhditis elegans genetic interactions, BioGRID data sets (Human, Saccharomyces cerevisiae , Drosphila and Mus musculus ), the internet (Autonomous Systems Level), and the US Power Grid. All the networks had many symmetries ranging in number from on the order of 10 13 to 10 11,298 , and could be decomposed into many subgroups (from 3 to more than 50). The subgroups were 90% or more made up of basic factors (not intertwined) consisting of various orders n of the symmetric group S n . Hence, viewed as dynamical networks, all could show ID in the right situations. The phenomena of symmetry-induced CS and ID appear to be possible in many model, man-made and natural networks, at least when modelled as unweighted couplings and identical systems. This is because our work here and that of refs 28 , 29 show that many types of networks can have symmetries and refs 20 , 21 show that many man-made and natural networks have dynamics similar to or reducible to equation (1) or its generalizations mentioned above. We have shown that ID is explained generally as a manifestation of clusters and subgroup decompositions. Furthermore, computational group theory can greatly aid in identifying CS in complex networks where symmetries are not obvious or far too numerous for visual identification. It also enables explanation of types of desynchronization patterns and transformation of dynamic equations into more tractable forms. This leads to an encompassing of or overlap with other phenomena, which are usually presented as separate. This list includes (1) remote synchronization [13] in which nodes not directly connected by edges can synchronize (this is just a version of CS), (2) some types of chimera states [27] , [37] , which can appear when the number of trivial clusters is large and the number of non-trivial clusters is small, but the clusters are big (see ref. 38 for some simple examples), (3) partial synchronization where only part of the network is synchronized (shown for some special cases in ref. 39 ). We note that although we have concentrated mostly on the maximal symmetry case, we can also examine the cases of lower symmetry induced by bifurcations that break the original symmetry and the same group theory techniques will apply to those cases. Some of this is developed for simple situations (rings or simple networks with point group symmetry) in ref. 15 , but we now have the ability to extend this to arbitrary complex networks. Calculating the IRR transformation Below are the steps necessary to determine the symmetries of the network, obtain the clusters, find the IRRs and, the most crucial part, calculate the transformation T from the node coordinates to the IRR coordinates that will block diagonalized A , as A commutes with all symmetries of the group [40] . Using the discrete algebra software, it is straightforward to determine the group of symmetries of A , extract the orbits that give the nodes in each cluster and extract the permutation matrices R g , and use the character table of the group and the traces of the R g ’s to determine which IRRs are present in the node-space representation of the group. Remark: this step is discussed in any book on representations of finite groups (for example, ref. 22 ). After this, we put each R g into its appropriate conjugacy class. To generate the transformaion T from the group information, we have written a code [41] on top of the discrete algebra software, which for each IRR present constructs the projection operator P (l) (ref. 22 ) from the node coordinates onto the subspace of that IRR, where l indexes the set of IRRs present. This is done by calculating, where is a conjugacy class, that is, α (l) the character of that class for the l th IRR, d (l) is the dimension of the lth IRR and is the order (size) of the group. Remark: the trivial representation (all IRR matrices=1 and α (l) =1) is always present and is associated with the synchronization manifold. All other IRRs are associated with transverse directions. Next we use singular value decomposition on P ( l ) to find the basis for the projection subspace for the l th IRR. Finally, we construct T by stacking the row basis vectors of all the IRRs, which will form an N × N matrix. We show the results of this applied to the 32-symmetry case in Fig. 1 : The non-trivial clusters are the nodes [1, 8], [2, 3, 7, 9], [4, 6], [5, 10] (the numbering of nodes matches the row and column numbers of A ). The transformation matrix is and the block diagonal coupling matrix is Experimental methods The SLM (Boulder Nonlinear Systems P512-1550) has an active area of 7.68 × 7.68 mm 2 and a resolution of 512 × 512 pixels. The camera (Goodrich SU320KTSW-1.7RT/RS170) has an indium gallium arsenide focal plane array with 320 × 256 pixels and an area of 8 × 6.4 mm 2 . Using a lens assembly, the SLM was imaged onto the camera with the magnification and orientation adjusted so that each 2 × 2 pixel area on the SLM is projected onto a camera pixel. The camera’s frame rate was ∼ 8 Hz and was synchronized with the SLM’s refresh rate. Each oscillator in equation (5) corresponds to a square patch of 16 × 16 pixels on the SLM, which is imaged onto an 8 × 8 pixel region of the camera’s focal plane array. The intensity ( x ) is the average of camera pixel values in this area. The same phase shift x is applied by each of the SLM pixels in the patch. We employ a spatial calibration and lookup table to compensate for inhomogeneities in the SLM. Data analysis methods The phase shifts imparted by each oscillator are recorded and used to determine the degree of synchronization, as shown in Fig. 3 . An individual oscillator’s deviation from synchronization at a given time as shown in Fig. 3c–e is measured by , where denotes a spatial average of the phases of all of the nodes within a particular cluster at time t . To quantify the degree of synchronization within a cluster as shown in Fig. 3a , we calculate the root-mean square synchronization error where ‹·› T indicates an average over a time interval T (here taken to be 500 iterations). How to cite this article: Pecora, L. M. et al . Cluster synchronization and isolated desynchronization in complex networks with symmetries. Nat. Commun. 5:4079 doi: 10.1038/ncomms5079 (2014).